Ultrafast spin-transfer torque driven by femtosecond pulsed-laser excitation Spin currents have an important role in many proposed spintronic devices, as they govern the switching process of magnetic bits in random access memories or drive domain wall motion in magnetic shift registers. The generation of these spin currents has to be fast and energy efficient for realization of these envisioned devices. Recently it has been shown that femtosecond pulsed-laser excitation of thin magnetic films creates intense and ultrafast spin currents. Here we utilize this method to change the orientation of the magnetization in a magnetic bilayer by spin-transfer torque on sub-picosecond timescales. By analysing the dynamics of the magnetic bilayer after laser excitation, the rich physics governing ultrafast spin-transfer torque are elucidated opening up new pathways to ultrafast magnetization reversal, but also providing a new method to quantify optically induced spin currents generated on femtosecond timescales. Ever since the discovery of the giant magnetoresistance effect by Fert and Grünberg [1] , [2] , spin-dependent transport phenomena have received growing attention due to the prospect of improving the efficiency and functionality of electronic devices by exploiting the electron spin [3] . A prime example of such a spintronic device is the spin-transfer torque (STT) magnetic random access memory, where a spin current is used to exert a torque on a magnetic bit ultimately switching its direction [4] , [5] , [6] , [7] , [8] . Recently, various novel schemes of STT switching have been proposed and demonstrated in the literature, ranging from using the spin-orbit interaction [9] , [10] , [11] or thermal gradients [12] , [13] , [14] , [15] , [16] , [17] , [18] to create spin currents and subsequently switch magnetic bits. A fascinating new approach to generate large spin currents on extremely short timescales is femtosecond (fs) pulsed-laser excitation of ferromagnetic thin films [19] , [20] . On absorption of a fs laser pulse, hot electrons are created that travel at high velocities and over tens of nanometers through the films. Because in a ferromagnet the lifetimes and velocities of excited majority and minority electrons differ, mobile majority electrons leave the ferromagnetic thin film after excitation leading to superdiffusive spin currents on fs timescales. Furthermore, the absorption of the laser pulse leads to huge thermal gradients, which also induce spin currents due to the spin or spin-dependent Seebeck effect [12] , [13] , [14] , [15] , [16] , [17] , [18] . Although the role these spin currents have in ultrafast demagnetization is being heavily debated [21] , [22] , the fact that laser-induced spin currents are present has been confirmed by several studies where the magnitude of the magnetization in a ferromagnetic layer is altered [23] , [24] , [25] , [26] , [27] , [28] , [29] , [30] . However, to ultimately switch a magnetic bit, it is crucial to actually change the orientation of the magnetic layer, that is, a torque has to be applied. Applying a torque with a fs laser pulse to the magnetization, and thus changing its orientation, has already shown to be possible by, for example, the inverse Faraday effect [31] . In the following, we will instead utilize fs laser-generated spin currents to control the orientation of the magnetization. In this Article, we first focus on experimentally demonstrating laser-induced STT on unprecedented timescales. Hereafter, we will discuss which of the proposed mechanisms are most likely to explain the experimental observations. Outline of the experiments The basic concept of our experiments is explained in Fig. 1 . 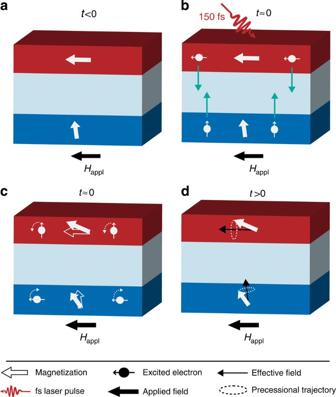Figure 1: Basic concept of the measurements to investigate pulsed laser-driven STT. A description of the used symbols is given at the bottom of the image. (a) Non-collinear magnetic bilayer before pulsed laser excitation. (b) Excitation of the bilayer by a fs laser pulse, resulting in angular momentum transfer between the two layers. (c) Change of the orientation of the magnetization in both layers due to the STT excerted by the excited electrons. (d) Precessional motion back to equilibrium after the STT pulse. Figure 1a displays the used non-collinear bilayer, which consists of an in-plane (IP) and an out-of-plane (OOP) magnetized film seperated by a non-magnetic spacer. During the experiments, a small IP magnetic field H appl is applied (black arrow), fixing the direction of the magnetization M (white arrow) of the IP film. Figure 1: Basic concept of the measurements to investigate pulsed laser-driven STT. A description of the used symbols is given at the bottom of the image. ( a ) Non-collinear magnetic bilayer before pulsed laser excitation. ( b ) Excitation of the bilayer by a fs laser pulse, resulting in angular momentum transfer between the two layers. ( c ) Change of the orientation of the magnetization in both layers due to the STT excerted by the excited electrons. ( d ) Precessional motion back to equilibrium after the STT pulse. Full size image Figure 1b shows the initial response of the magnetic bilayer to laser excitation. The laser pulse excites conduction electrons throughout the whole stack and creates large thermal gradients, leading to an IP spin current from top to bottom and an OOP spin current from bottom to top. When these spin-polarized conduction electrons reach the neighbouring magnetic layer, as shown in Fig. 1c , their transverse angular momentum is absorbed almost instantly by the local magnetization [32] , [33] , leading to an STT on the magnetic layer. The STT pulse thus changes the orientation of M away from the original equilibrium direction. This means that after excitation the magnetization does no longer point along the effective magnetic field H eff , and will start a damped precessional motion around this field, as depicted in Fig. 1d . The characteristics of the precession, such as its amplitude, frequency and phase, contain information on the excitation mechanism, and can thus be used to distinguish between ultrafast STT or other effects (see also Supplementary Note 1 , Supplementary Figs 1 and 2 and Supplementary Table 1 ). Furthermore, changing the direction of one of the layers switches the polarization of the generated spin currents, and hereby also the precessional phase, again allowing for the identification of ultrafast STT. Therefore, we will examine the laser-induced precessional dynamics for different configurations, applied fields and spacer materials to reveal the presence of ultrafast STT in the non-collinear bilayer. Sample structure and characterization For the measurements presented in this article samples are used, where the numbers represent the layer thicknesses in nm. A schematic overview of the sample is displayed in Fig. 2a . The bottom Pt layer is required for inducing the perpendicular anisotropy in the Co/Ni multilayer [34] , and the top Pt layer prevents oxidation of the sample. X (=Cu,Pt) is the spacer layer material with thickness d spacer . 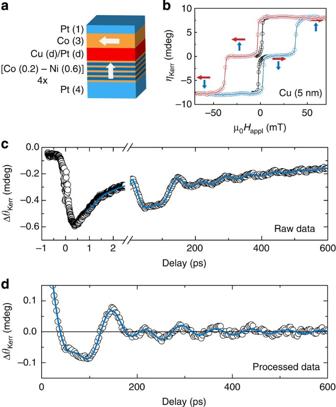Figure 2: Sample characteristics and data processing. (a) Structure used to investigate ultrafast STT. An IP magnetized Co film and a Cu or Pt spacer layer are deposited on a perpendicularly magnetized Co/Ni multilayer. (b) Longitudinal MOKE measurements for a 5-nm Cu spacer layer while applying an external field at an angle of 30°with respect to the film plane. The black lines denote the inner loops, revealing four stable configurations at zero field. (c) Typical time-resolved measurement forHappl=150 mT, fitted with a phenomenological function (see Methods). (d) Same data after removing the thermal background. Figure 2: Sample characteristics and data processing. ( a ) Structure used to investigate ultrafast STT. An IP magnetized Co film and a Cu or Pt spacer layer are deposited on a perpendicularly magnetized Co/Ni multilayer. ( b ) Longitudinal MOKE measurements for a 5-nm Cu spacer layer while applying an external field at an angle of 30 ° with respect to the film plane. The black lines denote the inner loops, revealing four stable configurations at zero field. ( c ) Typical time-resolved measurement for H appl =150 mT, fitted with a phenomenological function (see Methods). ( d ) Same data after removing the thermal background. Full size image Before performing any time-resolved measurements, the static magnetic properties of the fabricated samples were investigated by means of the magneto-optical Kerr effect (MOKE) with the probe laser at an incidence of 45°. A typical hysteresis loop is shown in Fig. 2b , where the normalized Kerr ellipticity η Kerr is plotted as a function of H appl for a Cu spacer layer thickness of 5 nm. H appl was rotated 30° with respect to the film plane to reverse both layers. Due to the relatively small spacer layer thickness (5 nm) with respect to the laser penetration depth (20 nm), both the bottom and the top layer of the film are probed simultaneously. The measurements clearly show two independently switching layers, where the film with the small (large) coercivity is the IP (OOP) film. The minimum values of d spacer for complete decoupling were determined to be 2 nm and 4 nm for Cu and Pt, respectively. Furthermore, four different remanent states at zero field can be distinguished, as indicated by the arrows in the image. Typical time-resolved MOKE measurements In the remainder of this article, we will address the time-dependent response of the magnetic bilayer to fs laser-pulse excitation. To measure M as a function of time, a time-resolved MOKE (TR-MOKE) setup is used (see Methods) in the polar MOKE geometry, hence the OOP component of M is measured. As we are solely interested in the precessional dynamics, demagnetization and subsequent remagnetization traces have been subtracted from the raw data before presentation. This is accomplished by fitting the data with a phenomenological fit function (see Methods), isolating the (damped) precessional motion sin( ωt + φ ). Typical values for the fit parameters can be found in Supplementary Table 2 . Before each measurement, the direction of the OOP film is set by applying a field perpendicular to the film plane. During the measurements, H appl is applied parallel to the film plane, which determines the orientation of the IP layer. Note that this IP field can trigger a precession of the OOP film, even in the absence of any spin currents. The origin of this precession is a sudden change in the anisotropy Δ K on pulsed laser heating, resulting in a change of the direction of H eff (ref. 35 ). Therefore, care has to be taken on analysing the dynamics of the OOP film. The IP film cannot be excited by this mechanism since the external field is applied along an easy axis, hence the direction of H eff is not changed by the laser pulse. Therefore, the main conclusions in this article will be drawn from the observed precession of the IP film. A typical time-resolved measurement is depicted in Fig. 2c , where the laser-induced change in the Kerr angle Δ θ Kerr is plotted as a function of time delay. After pulsed laser excitation, the OOP layer shows a rapid demagnetization in 300 fs, followed by a remagnetization on a ps timescale. The signal is coming from the OOP layer, since the longitudinal dynamics of the IP layer cannot be observed in the polar MOKE geometry. On a longer timescale, two effects are observed. First, the magnetization relaxes back towards equilibrium due to heat diffusion to the substrate. More importantly, two precessions can be distinguished with different precession frequencies, indicating that a precession is induced in both the IP and OOP layer. To extract the precessional motion, the thermal background is removed by fitting the data after 1 ps with a phenomenological fitting function (see Methods). The result is depicted in Fig. 2d clearly revealing the two precession. Precessional motion for the four configurations We start our investigation of ultrafast STT by measuring the laser-induced precessions for the four different configurations depicted in Fig. 2b . This is motivated by the notion that the expected precessional phase of the IP layer depends on the orientation of the OOP layer, simply because the latter influences the sign of the generated spin current. For the Δ K mechanism, no change of the phase of the IP layer is expected on switching the OOP layer. The measurements for a Cu spacer ( d spacer =5 nm) and H appl =70 mT are displayed in Fig. 3 , where the lines are fits with two exponentially damped sines. The data and fits clearly reveal two precessions with different frequencies, of which the individual contributions are drawn as lines in the top panel of Fig. 3 for one configuration of the bilayer. We attribute the high-frequency long-lived precession to the IP layer, while the low-frequency highly damped precession originates from the OOP layer. This assumption will further on be verified by analysing the precession frequencies as a function of H appl , which show a distinctly different behaviour for the IP and OOP layer. The most important conclusion from Fig. 3 is that the precessional phase of the IP layer is solely determined by the orientation of the OOP layer, which is fully consistent with our expectations of an ultrafast laser-induced STT. Furthermore, this excludes that the precession of the IP layer is caused by the Δ K mechanism or any other mechanism in which only one of the layers is involved, for example, magnetostrictive effects [36] . 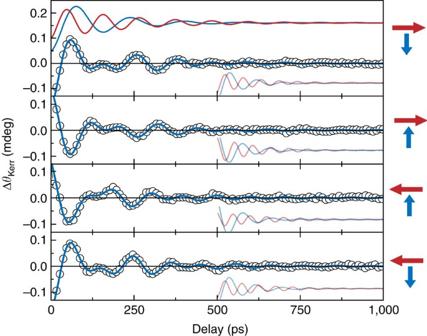Figure 3: Time-resolved measurements of the OOP component of the magnetization for the four different configurations of the bilayer. The Kerr rotationθKerris plotted as a function of delay time after pulsed laser excitation for the magnetic bilayer withdCu=5 nm, while applying an IP magnetic fieldHapplof 70 mT. For clarity, the thermal background has been subtracted from the raw data. In the top graph also the two fitted precessions are plotted, which are also shown as transparent lines in the bottom-right corner of every panel. Note that, for the latter, the axes have been rescaled for clarity. Figure 3: Time-resolved measurements of the OOP component of the magnetization for the four different configurations of the bilayer. The Kerr rotation θ Kerr is plotted as a function of delay time after pulsed laser excitation for the magnetic bilayer with d Cu =5 nm, while applying an IP magnetic field H appl of 70 mT. For clarity, the thermal background has been subtracted from the raw data. In the top graph also the two fitted precessions are plotted, which are also shown as transparent lines in the bottom-right corner of every panel. Note that, for the latter, the axes have been rescaled for clarity. Full size image Influence of spacer layer thickness and material We now continue by comparing the laser-induced magnetization dynamics between a sample with a Cu spacer and a Pt spacer. For the Cu spacer, we expect that the created spin currents can reach the adjecent magnetic layer, as schematically depicted in Fig. 4a . However, for the strong spin scatterer Pt, the spin current is most likely severely attenuated by spin-flip scattering, as shown by Fig. 4b , resulting in a heavily reduced precessional amplitude. In case of the Cu spacer layer, again two precessions are visible in the data. However, Fig. 4d shows that only the precession of the OOP layer is visible in case of a Pt spacer layer, meaning that the other precession is quenched. We attribute this to a reduced spin current flow between the layers, indicating that the oscillations of the IP layer seen in Fig. 4c are caused by a fs laser-induced spin transfer. On the other hand, this also means that the precessions of the OOP layer have a different origin, which is most likely the aforementioned Δ K mechanism. Note that, thus, also the precession amplitudes for the Pt and Cu spacer layer are of roughly the same magnitude in the OOP layer. In Fig. 1d , it was shown that an STT pulse should, in principle, also induce a precession in the OOP layer; however, we have calculated that the expected STT effects to the magneto-optical signal should be relatively small (see Supplementary Note 2 and Supplementary Figs 3–5 ), and thereby easily overwhelmed by the Δ K mechanism. 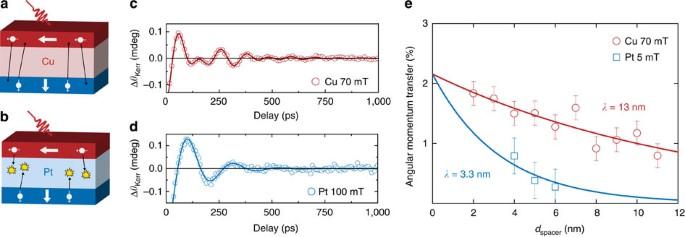Figure 4: Spacer layer dependence of the laser-induced precessions. (a) Angular momentum exchange between the IP and OOP layer through a Cu spacer layer. (b) Spin scattering in Pt, suppressing the exchange of angular momentum. OOP precessional dynamics of a Cu (c) and Pt (d) spacer layer of 5-nm thick, revealing that the Pt spacer layer quenches the precessional motion of one of the layers. The lines are fits with a phenomenological fit function (see Methods). (e) Percentage of spins participating in the demagnetization of the OOP layer that are absorbed by the IP layer as a function of spacer layer thickness, as deduced from measurements at 25 mT (Cu) and 5 mT (Pt). The error bars are determined from the fits of the static and dynamics measurements. Figure 4: Spacer layer dependence of the laser-induced precessions. ( a ) Angular momentum exchange between the IP and OOP layer through a Cu spacer layer. ( b ) Spin scattering in Pt, suppressing the exchange of angular momentum. OOP precessional dynamics of a Cu ( c ) and Pt ( d ) spacer layer of 5-nm thick, revealing that the Pt spacer layer quenches the precessional motion of one of the layers. The lines are fits with a phenomenological fit function (see Methods). ( e ) Percentage of spins participating in the demagnetization of the OOP layer that are absorbed by the IP layer as a function of spacer layer thickness, as deduced from measurements at 25 mT (Cu) and 5 mT (Pt). The error bars are determined from the fits of the static and dynamics measurements. Full size image We will now proceed to quantify the amount of spin transport as a function of Cu and Pt spacer layer thickness. To this extent, time-resolved measurements were performed as a function of d spacer for both Cu and Pt spacer layers. The precession amplitudes were obtained by fitting the time-resolved traces, like in Fig. 4c,d . From the fitted amplitudes, a canting angle of 60 mdeg was obtained for d Cu =5 nm ( Supplementary Note 3 and Supplementary Fig. 6 ). From the fits, the amount of angular momentum transferred from the OOP to the IP layer is calculated as a fraction of the angular momentum lost due to demagnetization of the OOP layer ( Supplementary Note 3 ). The results are depicted in Fig. 4e . Note that for the Pt spacer layer, a much smaller field was applied during the measurements to reduce the precessions caused by the Δ K mechanism. As expected, the angular momentum transfer shows a decrease on increasing d Cu or d Pt . By fitting the data with an exponential decay, the spin-transfer length λ is determined for both layers. The fits, depicted as lines in Fig. 4e , yield λ Cu =13±3 nm and λ Pt =3.3±0.4 nm showing that indeed the spin-transfer length in a strong spin scatterer like Pt is limited. Finally, we would like to note that for large values of λ , there is no strict correspondence to the spin diffusion length as measured in transport studies, because the present work focusses on highly excited (‘hot’) electrons. Field and angle dependence of precession characteristics As already mentioned, the frequencies, amplitudes and phases of the precessions reveal information on the type of excitation mechanism, but also on its duration d pulse (see Supplementary Note 1 ). Therefore, the precessional frequencies, amplitudes and phases are measured as a function of both the magnitude and direction of H appl in the samples with a 5-nm Cu spacer layer. By comparing the results to expectations based on macro-spin calculations, we can verify that indeed the precession in the IP layer is caused by a short spin current pulse, and the precession in the OOP layer by a change in anisotropy Δ K . The results for the configuration where the OOP layer is pointing downwards (− z direction) are depicted in Fig. 5 . 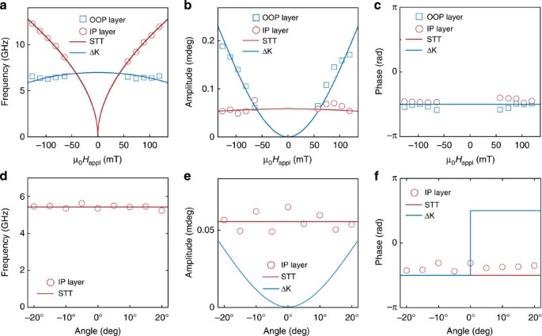Figure 5: Detailed investigation of precessional characteristics. The precession frequency, amplitude and phase of the IP and OOP layer fordCu=5 nm are measured as a function of the magnitude and direction ofHappl. All the data are obtained by fitting the raw TR-MOKE traces with a phenomenological fitting function. In the measurements where the applied field strength is varied, that is, (a–c), the field is applied at an angle of 0° with respect to the film plane, whereas the angle-dependent measurements (d–f) are performed for a field strength of 25 mT. The solid lines inaare fits to analytical expressions derived from the Landau–Lifschitz–Gilbert equation (see main text), and the solid lines inb–fare calculated using a macro-spin model with an ultrafast STT pulse or a step-like change in the anisotropy ΔKfor the IP layer and a step-like change in the anisotropy ΔKfor the OOP layer. Figure 5: Detailed investigation of precessional characteristics. The precession frequency, amplitude and phase of the IP and OOP layer for d Cu =5 nm are measured as a function of the magnitude and direction of H appl . All the data are obtained by fitting the raw TR-MOKE traces with a phenomenological fitting function. In the measurements where the applied field strength is varied, that is, ( a – c ), the field is applied at an angle of 0° with respect to the film plane, whereas the angle-dependent measurements ( d – f ) are performed for a field strength of 25 mT. The solid lines in a are fits to analytical expressions derived from the Landau–Lifschitz–Gilbert equation (see main text), and the solid lines in b – f are calculated using a macro-spin model with an ultrafast STT pulse or a step-like change in the anisotropy Δ K for the IP layer and a step-like change in the anisotropy Δ K for the OOP layer. Full size image Figure 5a shows the fitted precession frequencies as a function of μ 0 H appl . For μ 0 H appl <50 mT, the two precessions could not be separated, hence the lack of data points in this region. For larger values of the field, the data points for the IP and OOP layer can be easilly separated due to their distinctly different field dependence: the IP layer follows the Kittel relation (ref. 37 ), whereas the OOP layer is governed by (ref. 38 ), with H K being the effective perpendicular anisotropy field. The lines in Fig. 4a are fits of the data to these relations and result in a value of 1.1 × 10 6 A m −1 for M sat of the IP Co layer, which is reasonable compared with the bulk value of 1.4 × 10 6 A m −1 and μ 0 H K of 250 mT. The amplitude and phase of both precessions are plotted as a function of the magnitude of H appl in Fig. 5b,c , respectively, where the lines in the graphs correspond to macro-spin calculations. Unlike in the case for the frequency, no analytical solution can be obtained as details of the spin current pulse determine the amplitude and phase of the precession. In the calculations, it is assumed that the IP layer is excited by a very short STT pulse, such that t pulse <<2 π / ω . Furthermore, it is assumed that the OOP layer is excited by a step-like decrease in the anisotopy Δ K . The excellent agreement between the measurements and the calculations validate these assumptions. Next, measurements on the IP layer, where the angle of H appl is varied, are compared with macro-spin calculations in Fig. 5d–f . Again, assuming excitation by a short STT pulse yields good correspondence to the data, verifying that the orientation of the IP is changed by ultrafast laser-induced spin currents. Based on Fig. 5e,f , the Δ K mechanism can again be ruled out as the origin of the precession of the IP layer due to the completely different angle dependence of the precessional amplitude and phase. For the calculation, a step-like change in the anisotropy is assumed on pulsed laser excitation, as this gives closest correspondence to the experimentally observed phase. It has already been mentioned that the observed spin currents can potentially be generated by both superdiffusive transport and spin Seebeck-like effects. Further, we will discuss whether these mechanisms are likely to account for the experimentally observed ultrafast transfer of angular momentum. We first turn our attention to superdiffusive transport [19] , [20] , as this theory has experimentally been shown to apply to the here performed experiments, that is, fs laser-pulse excitation of magnetic multilayers [25] , [28] , [29] . From the magnitude of the spin transfer in Fig. 4e , it can be concluded that superdiffusive spin currents provide a realistic scenario for the observed ultrafast STT. Only ≈2% of the spins participating in the demagnetization of the OOP layer are transferred to the IP layer, indeed not exceeding the theoretical predictions [19] and experimental observations [21] , [23] , [25] , where 10–100% of the demagnetization is caused by spin currents. Next to superdiffusive spin currents due to hot non-equilibrium electrons, the presence of thermal gradients after fs pulsed-laser excitation could lead to spin Seebeck-like effects. In the literature, different types of spin Seebeck effects have been proposed, originating from temperature differences at magnetic/non-magnetic interfaces [12] , magnon-driven spin currents due to a bulk temperature gradient [13] , [18] or spin-dependent Seebeck coefficients combined with temperature gradients within the magnetic thin films [14] , [15] , [39] . The magnonic or spin-wave-like effects appear to be dominant on long lengthscales (several micro- to millimeters) or in magnetic insulators, whereas the interface effects have shown to be too weak to explain experimental data on similar structures (metallic magnetic multilayers) as used in the present experiments [14] . Although contribution from both these effects cannot be completely excluded under the strong non-equilibrium condition investigated here, we will focus on the spin-dependent Seebeck effect, that is, the generated spin current due to different Seebeck coefficients of majority and minority electrons. We first performed simulations of the dynamical temperature profile to calculate the temperature gradients present during the experiments. These temperature gradients are used as input for a simple drift-diffusion model to calculate the spin-dependent Seebeck currents, from which the amplitude and phase of the induced precessions can be deduced. Details of the calculations can be found in Supplementary Note 4 and Supplementary Figs 7–10 , and show that the spin-dependent Seebeck effect is over an order of magnitude too weak to explain the experimental observations. In principle, the phase of the precession can be used to distinguish the spin Seebeck contributions from superdiffusive spin currents. However, unfortunately, the analysis shows that in the present case the difference is too small to separate them within the uncertainty margins. Finally, we rule out magnetostatic coupling, being either an exchange [40] , [41] or dipolar (Néel) coupling [42] , as the mechanism that could have induced the precessions in the measurements. Both coupling mechanisms contribute to H eff , and depend linearly on M of the neighbouring layer. As pulsed laser excitation induces a change in the magnetization Δ M on ultrafast timescales, it hereby also affects H eff . However, based on estimates of the required coupling strengths and the dependence of the precession amplitude on the spacer layer thickness and material, it can be concluded that magnetostatic coupling cannot explain the induced precessions ( Supplementary Note 5 ). Altogether, the observed fs STT can unambiguously be assigned to superdiffusive spin currents generated by ultrashort intense laser pulses. In conclusion, we have experimentally demonstrated that spin currents generated by pulsed laser excitation can tilt the magnetization of a thin magnetic film away from its equilibrium direction, launching precessional motion of the IP film of a non-collinear magnetic bilayer. This allows for control of the direction of the local magnetization on unprecedented timescales. By careful analysis of the experimental data, superdiffusive spin currents have been identified as the main contributor to the observed STT. The control of the orientation of the magnetization in thin films by superdiffusive spin currents could potentially be used for all-optical switching of the magnetization in future magnetic storage devices. Furthermore, the here presented experiments on a non-collinear bilayer provide an accurate probe for the amount of angular momentum transfered on ultrafast laser heating, contributing to the recent debate on the competition between spin-flip scattering and spin transport as a driving force for ultrafast demagnetization. Time-resolved measurements The dynamics of the magnetic bilayer after pulsed laser excitation were studied with a TR-MOKE setup in the polar MOKE geometry, where a pump and probe beam from an 80 MHz Ti:sapphire laser with a wavelength of 790 nm and pulse length of 150 fs are focussed to an 8 μm diameter spot. The sample is both excited as probed from the top side of the sample. Before each measurement, the orientation of the magnetization in the OOP layer is set by applying a positive or negative field in the perpendicular ( z ) direction. During the measurement, an IP field is applied to fix the orientation of the IP layer. Data analysis To analyse the precessional data quantitatively, all TR-MOKE remagnetization traces are fitted with the following phenomenological function: where t is the delay time between arrival of the probe pulse with respect to the probe. The first term is an offset due to direct current heating of the sample, the second term represents remagnetization due to electron–phonon equilibration, the third and fourth term represent model cooling due to heat flow through a thin insulating layer into the substrate. The fifth and sixth term resemble the precessions of the IP and OOP layers, where t d is the typical timescale for the damping, ω is the angular velocity of the precession and φ is the phase. All constants are used as fitting parameters. Macro-spin simulations For the calculations on the induced precessional dynamics, the following form of the Landau–Lifschitz–Gilbert equation is used: where m is the normalized magnetization M / M , γ is the gyromagnetic ratio, α is the Gilbert damping constant, J s is the spin current density, d is the thickness of the magnetic thin film, and σ is the unit vector along the polarization direction of the spin current. Both J s and H eff are time dependent due to excitation by the laser pulse. In the calculations, σ points along M OOP for the IP layer and vice versa. Material parameters used in the calculations are 0.02 and 0.2 for the damping constants and M sat =1,400 A m −1 and 776 A m −1 for the IP and OOP films, respectively. Furthermore, H eff consists of two contributions, being the applied field H appl and the anisotropy field H K , which is equal to for the IP and for the OOP layer. How to cite this article : Schellekens, A. J. et al. Ultrafast spin-transfer torque driven by femtosecond pulsed-laser excitation. Nat. Commun. 5:4333 doi: 10.1038/ncomms5333 (2014).